Plasmonic gold mushroom arrays with refractive index sensing figures of merit approaching the theoretical limit Localized surface plasmon resonance (LSPR)-based sensing has found wide applications in medical diagnosis, food safety regulation and environmental monitoring. Compared with commercial propagating surface plasmon resonance (PSPR)-based sensors, LSPR ones are simple, cost-effective and suitable for measuring local refractive index changes. However, the figure of merit (FOM) values of LSPR sensors are generally 1–2 orders of magnitude smaller than those of PSPR ones, preventing the widespread use of LSPR sensors. Here we describe an array of submicrometer gold mushrooms with a FOM reaching ~108, which is comparable to the theoretically predicted upper limit for standard PSPR sensors. Such a high FOM arises from the interference between Wood’s anomaly and the LSPRs. We further demonstrate the array as a biosensor for detecting cytochrome c and alpha-fetoprotein, with their detection limits down to 200 pM and 15 ng ml −1 , respectively, suggesting that the array is a promising candidate for label-free biomedical sensing. Localized surface plasmon resonances (LSPRs) carried by noble metal nanocrystals and nanostructures can concentrate light into nanoscale spatial regions, which enables many important applications, such as sunlight harvesting [1] , surface-enhanced Raman scattering [2] and sensing [3] . Compared with commercially available sensors based on propagating surface plasmon resonances (PSPRs), LSPR sensors are simple, cost-effective and suitable for measuring local refractive index changes caused by the adsorption of target molecules [4] , [5] , [6] . However, the figure of merit (FOM) values, which are refractive index sensitivities divided by plasmon resonance linewidths, of LSPR sensors are generally 1–2 orders of magnitude smaller than those based on PSPRs ( Supplementary Tables S1 and S2 ). Owing to strong radiative damping, the LSPRs of metal nanostructures generally exhibit broad resonance peaks, which result in small FOM values and in turn limit the performances of LSPR sensors [7] , [8] , [9] . To increase the FOM of a LSPR sensor, one can increase its index sensitivity and/or reduce the full width at half maximum (FWHM) of the LSPR. By lifting metal nanostructures above substrates with dielectric pillars, the index sensitivity of the resultant LSPR sensors can be increased because a large fraction of the spatial region with enhanced electric fields is exposed to the environment and accessible by molecular species [10] , [11] . More efforts have been made to reduce the FWHM values of LSPRs and therefore increase the FOM values [12] , [13] , [14] , [15] , [16] , [17] , [18] , [19] , [20] , [21] , [22] , [23] , [24] , [25] , [26] , [27] , [28] . An effective approach for reducing the FWHM values is to couple a LSPR with a different resonance mode that possesses a smaller FWHM. Split ring resonator-bar structures [12] , lifted cross-bar structures [13] , closely packed nanodisk clusters [14] and silver nanocubes supported on dielectric substrates [8] have been shown to possess high FOM values because of the occurrence of Fano resonances arising from the coupling between broad superradiant and narrow subradiant modes. The coupling of a plasmonic nanocube with a dielectric substrate [16] can be optimized to give a FOM of 12–20. Another scheme for decreasing plasmonic FWHM values is to pattern metal nanoparticles into one- or two-dimensional arrays [17] , [18] , [19] , [20] , [21] . The diffractive coupling among periodically arranged metal nanoparticles has been shown to give lattice plasmon resonances with FWHM values below 10 nm (refs 19 , 20 , 21 ). In addition, the FWHM and sensing capability of LSPRs can also be improved by coupling them with photonic microcavities [22] , [23] , [24] , [25] . Apart from monitoring the spectral shifts caused by small changes in the refractive index of the local surrounding environment, intensities [26] and phases [27] have also been examined to improve the sensing performance of LSPR sensors. Despite the aforementioned efforts, the FOM values of LSPR sensors have still remained uncompetitive with those of PSPR sensors ( Supplementary Tables S1 and S2 ), which severely restricts the practical applications of LSPR sensors. Here we describe the fabrication and characterization of a periodic array of gold mushrooms. Each mushroom is at the submicrometer scale and composed of a gold cap on a photoresist pillar, the bottom of which is located in a hole in a gold film. In this gold mushroom array (GMRA) structure, a new coupled plasmon resonance mode with a narrow FWHM (~10 nm or ~0.007 eV) and a high refractive index sensitivity (~1,010 nm RIU −1 ; refractive index unit) are simultaneously obtained. The resonance mode originates from the coupling of LSPRs with Wood’s anomaly (WA), the latter of which is caused by the diffraction of the incident light into a propagating wave, with its propagation direction being tangential to the grating surface. In contrast to PSPRs, the coupled resonance mode can be readily excited without the use of prisms or gratings to overcome the momentum mismatch problem. The combination of the narrow linewidth and high-index sensitivity gives rise to an unprecedented FOM, which is up to ~108. This FOM is comparable to the theoretically estimated upper FOM limit (~108) for standard PSPR sensors made of gold film under the Kretschmann configuration. In addition, a Rabi splitting-type anticrossing between WA and a Fabry–Pérot cavity mode is also observed. Further, biosensing based on the GMRA with detection limits down to 200 pM and 15 ng ml −1 is demonstrated for detecting cytochrome c (Cyt c ) and alpha-fetoprotein (AFP), respectively. GMRA fabrication The array structure ( Fig. 1a ) is constructed according to the consideration of increasing its FOM by simultaneously improving its refractive index sensitivity and reducing its FWHM. Specifically, gold caps are lifted by dielectric pillars with a small refractive index. As a result, more spatial regions around the gold caps with plasmon-enhanced electric fields will be accessible by the surrounding environment. Therefore, the apparent refractive index sensitivity of the lifted metal caps will be increased [10] . Moreover, a Fano resonance caused by the interference between WA of the periodic array and the LSPR of the individual gold units is simultaneously introduced. The presence of the Fano resonance results in a large reduction in the spectral linewidth. On the basis of the consideration above, we employed double two-beam interference lithography to pattern a periodic array of photoresist pillars in a square lattice, followed by thermal evaporation of gold to produce the GMRA ( Fig. 1a ). The photoresist pillars have a rounded square cross-section, and their height can be varied. The fabrication process involves only two major steps. It is simple and cost-effective, which is beneficial for practical sensing applications. 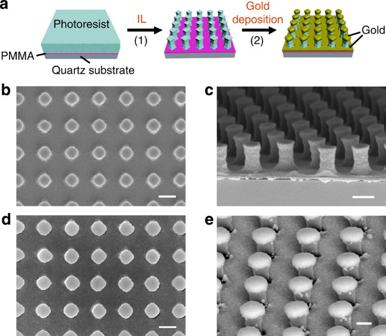Figure 1: GMRAs. (a) Schematic showing the fabrication procedure. PMMA refers to poly(methyl methacrylate). IL stands for interference lithography. (b,c) Top- and side-view SEM images of a periodic array of rounded square photoresist pillars (lattice constanta=610 nm, pillar heighth=510 nm). (d,e) Top- and side-view SEM images of the photoresist array deposited with gold. The side length of the gold cap on the pillar top and the hole in the bottom gold film isl=285 nm. The thickness of the gold layer ist=110 nm. The spacing between the bottom of the gold caps and the top of the gold film is therefore 400 nm. (b–d) Scale bars, 400 nm. (e) Scale bar, 200 nm. Figure 1b,c show the top- and side-view scanning electron microscopy (SEM) images of an array of photoresist pillars obtained after interference exposures and development. The pillars are nearly square. The top of each pillar is slightly larger than the middle, which is beneficial for the subsequent formation of a gold cap through thermal evaporation because the larger top can prevent gold deposition on the side of the pillar. Figure 1d,e show the top- and side-view SEM images of a GMRA. The gold caps are rounded and larger than the photoresist pillars. Almost no gold is observed on the side wall of the pillars. The entire structure looks like a periodic array of mushrooms grown on a gold film with a periodic array of holes. Figure 1: GMRAs. ( a ) Schematic showing the fabrication procedure. PMMA refers to poly(methyl methacrylate). IL stands for interference lithography. ( b , c ) Top- and side-view SEM images of a periodic array of rounded square photoresist pillars (lattice constant a =610 nm, pillar height h =510 nm). ( d , e ) Top- and side-view SEM images of the photoresist array deposited with gold. The side length of the gold cap on the pillar top and the hole in the bottom gold film is l =285 nm. The thickness of the gold layer is t =110 nm. The spacing between the bottom of the gold caps and the top of the gold film is therefore 400 nm. ( b – d ) Scale bars, 400 nm. ( e ) Scale bar, 200 nm. Full size image Resonance modes of the GMRA We measured the reflectance spectra of the GMRA at varying incidence angles with an s -polarized incident wave. The plane of incidence was along the Γ–X direction. The experimental zero-order reflectance spectrum at normal incidence in air is shown by the red curve in Fig. 2b . The black curve in this figure is the spectrum simulated by the finite-difference time-domain (FDTD) method. The simulated and experimental spectra agree well with each other in the prediction of the peak and dip positions. There are two peaks and two dips in the near-infrared region. The simulations show that the electric field distribution at P1 (879 nm) is localized around the diagonal corners of the gold cap ( Fig. 2d ), indicating that P1 is caused by the LSPR of the gold caps. We performed the FDTD simulations for the structure that contains a periodic array of the gold mushrooms but without the perforated gold film ( Fig. 2c ). The structure exhibits a strong peak P1′, which has nearly the same spectral position and field distribution ( Fig. 2h ) as P1, confirming that P1 is a LSPR arising from the gold caps. For the dip D4 (1,178 nm), the electric field is mainly distributed in the gold hole and on the gold cap ( Fig. 2g ). To identify D4, we also performed the simulations for the structure that contains the periodically positioned pillars and perforated gold film but without the gold caps ( Fig. 2a ). For this structure, there exists a dip D4′, which is caused by the LSPR of the gold holes, as revealed by the electric field distribution ( Fig. 2i ). Compared with D4′, D4 of the GMRA is pushed to a longer wavelength, which is believed to be caused by the LSPR of the gold caps. D4 can therefore be thought of arising from the interference between the LSPRs of the gold holes and caps. The dip D3 and peak P2 are ascribed to the interaction between the LSPRs of the gold cap array and perforated gold film. Specifically, the upper gold cap layer and lower perforated gold film layer form a Fabry–Pérot-type cavity, which gives rise to D3 and P2. The electric field distributions for D3 and P2 are found to concentrate at the gold cap and the side of the dielectric pillar ( Fig. 2e,f ). The strong coupling between the upper and lower layers is even more obvious at oblique incidence angles ( Supplementary Fig. S1 ). These Fabry–Pérot-derived dip and peak are similar to those described in a previous study [29] . 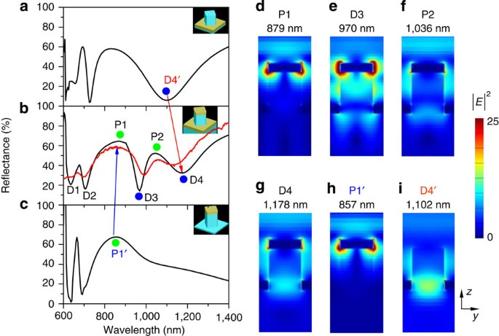Figure 2: Reflectance and electric field intensity distributions at normal incidence in air. (a) Simulated reflectance spectrum for the structure composed of only the photoresist pillars and perforated gold film. (b) Measured (red curve) and simulated (black curve) reflectance spectra for the GMRA (a=610 nm,h=510 nm,l=285 nm andt=110 nm). (c) Simulated reflectance spectrum for the structure composed of only the periodic array of the gold mushrooms but without the perforated gold film. The insets ina–cshow the schematics of the corresponding structures. The red arrow indicates that the dip D4 inband the dip D4′ inahave a similar origin, and the blue arrow indicates that the peak P1 inband the peak P1′ inchave the same origin. (d–i) Simulated electric field intensity distributions for the peaks and dips, respectively, at the linear scale. Figure 2: Reflectance and electric field intensity distributions at normal incidence in air. ( a ) Simulated reflectance spectrum for the structure composed of only the photoresist pillars and perforated gold film. ( b ) Measured (red curve) and simulated (black curve) reflectance spectra for the GMRA ( a =610 nm, h =510 nm, l =285 nm and t =110 nm). ( c ) Simulated reflectance spectrum for the structure composed of only the periodic array of the gold mushrooms but without the perforated gold film. The insets in a – c show the schematics of the corresponding structures. The red arrow indicates that the dip D4 in b and the dip D4′ in a have a similar origin, and the blue arrow indicates that the peak P1 in b and the peak P1′ in c have the same origin. ( d – i ) Simulated electric field intensity distributions for the peaks and dips, respectively, at the linear scale. Full size image In the visible spectral region, the reflectance spectrum of the GMRA at normal incidence exhibits two dips D1 (635 nm) and D2 (705 nm). D1 arises from (1, 0) WA, which is caused by the coupling of the incident light to a diffracted grazing wave in air [30] , [31] . D2 is attributed to the (1, 1) surface plasmon polariton (SPP) at the gold–PMMA interface. For a square lattice, the momentum-matching condition between these modes and the in-plane wavevectors of the incident light can be described by Bragg’s coupling equation [32] : where i and j are the grating orders for the reciprocal lattice vectors G x and G y (| G x |=| G y |=2 π / a , a is the lattice constant), θ is the incidence angle from air, k 0 is the wavevector of the incident light, and k mode is the wavevector of a specific mode (SPP or WA) of the structure. The wavevectors k spp and k WA of the SPP and WA modes are given by [33] , [34] : where ε m and ε d are the dielectric constants of the metal and surrounding medium, respectively. According to the three equations above, at normal incidence in air, the wavelengths of WA λ WA (1, 0) and the SPP mode λ SPP (1, 1) are calculated to be 610 and 700 nm, respectively. The calculated wavelengths are both in good agreement with the experimental ones, confirming that D1 and D2 originate from (1, 0) WA in air and the (1, 1) SPP mode at the gold–PMMA interface, respectively. WA has been known to shift with the incidence angle. In our case, (1, 0) WA red-shifts as the incidence angle is increased. In contrast, LSPRs are independent of the incidence angle. The two resonances are straightforwardly expected to eventually overlap to create a coupled resonance with a narrow FWHM if the incidence angle is increased. We therefore simulated (Fig. 3a) and measured (Fig. 3b) the reflectance spectra of the GMRA, as the incidence angle was varied from 8° to 36°. The overall trends revealed by the simulated reflectance spectra agree reasonably well with those by the experimental ones. D1, arising from (1, 0) WA, shifts to the longer-wavelength region as the incidence angle is increased (red dashed line in Fig. 3a), which is expected according to equations (1) and (3). As (1, 0) WA partially overlaps with the LSPR of the gold caps, D1 shows a Fano-like lineshape and is formed by the interference between (1, 0) WA and the scattered light from the gold caps. When the incidence angle is in the range of 25°–31°, as marked by the black dashed lines in Fig. 3a , a Rabi splitting-type anticrossing [35] , [36] between D1 and D3 is observed on both the simulated and measured reflectance spectra (see Supplementary Fig. S1 for the mode exchange details). The anticrossing suggests a strong coupling between the two different resonances, that is, WA and the Fabry–Pérot-type mode, the latter of which is caused by the interaction between the LSPRs of the gold cap array and perforated gold film. When the incidence angle is equal to 34°, as marked by the black dashed line in Fig. 3b , the FWHM of D1 is found to narrow down to 15.8 nm ( Fig. 3c ). Such a narrow FWHM suggests that D1 can be an excellent candidate for a refractive index sensor. We also checked the reflectance spectra recorded in air with the incidence angle varied from 36° to 68° ( Supplementary Fig. S2 ). As the incidence angle is increased, D4 decreases gradually in intensity and disappears finally. No anticrossing between D1 and D4 is observed. We further measured angle-resolved reflectance spectra of the GMRA ( Supplementary Fig. S3 ) under p -polarized incident light. As the reflectance spectra under p -polarized incident light do not show any sharp peaks or dips at any measured incidence angle, they are not suitable for sensing applications. In this study, we therefore only consider the reflectance spectra under s -polarized incident light. 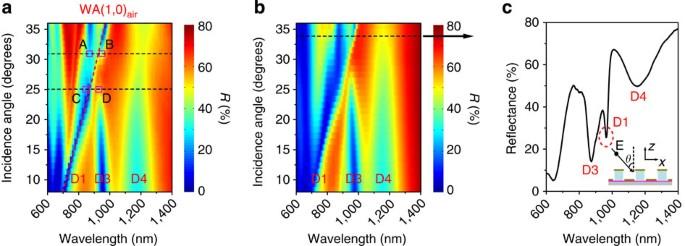Figure 3: Angle-resolved reflectance spectra of the GMRA in air. (a) Simulated and (b) measured reflectance spectra for the incidence angle varied from 8° to 36° at a step of 1°. The red dashed line inadenotes (1, 0) Wood’s anomaly (WA). There is a clear anticrossing between WA (D1) and the Fabry−Pérot-type mode (D3) marked by A, B, C and D ina, with the two black dashed lines denoting the incidence angles of 25° and 31°, respectively. (c) Experimental reflectance spectrum at the incidence angle of 34°, as indicated by the black dashed line inb. The inset incshows the reflectance measurement geometry. The red dotted ellipse indicates the sharp dip, which is highly desirable for sensing applications. The sizes of the GMRA area=610 nm,h=510 nm,l=285 nm andt=110 nm. Figure 3: Angle-resolved reflectance spectra of the GMRA in air. ( a ) Simulated and ( b ) measured reflectance spectra for the incidence angle varied from 8° to 36° at a step of 1°. The red dashed line in a denotes (1, 0) Wood’s anomaly (WA). There is a clear anticrossing between WA (D1) and the Fabry−Pérot-type mode (D3) marked by A, B, C and D in a , with the two black dashed lines denoting the incidence angles of 25° and 31°, respectively. ( c ) Experimental reflectance spectrum at the incidence angle of 34°, as indicated by the black dashed line in b . The inset in c shows the reflectance measurement geometry. The red dotted ellipse indicates the sharp dip, which is highly desirable for sensing applications. The sizes of the GMRA are a =610 nm, h =510 nm, l =285 nm and t =110 nm. Full size image FOM of the GMRA To examine the performance of the GMRA as a refractive index sensor, we measured the zero-order reflectance spectra at the incidence angle of 33.3° when the GMRA was immersed in glycerine–water mixture solutions with varying compositions and therefore different refractive indices ( Fig. 4a ). The dip around 1,420 nm is the absorption band of water. In the solutions, the red shift of D1 with increasing incidence angles causes a spectral overlapping of D1 with D4 and leads to the generation of a coupled WA–LSPR mode (see Discussion section below). To see clearly the spectral shift of D1 with the increase in the refractive index of the surrounding environment, we plotted the normalized reflectance spectra in the spectral range of 1,240–1,350 nm ( Fig. 4b ). The FWHM of D1 (see Supplementary Fig. S4 for the determination of the FWHM values) is in the range of 9.5 nm (0.0071, eV)–12.7 nm (0.0088, eV). The extremely narrow FWHM of 9.5 nm is obtained at λ =1,288 nm in the mixture solution containing 25.96 wt% glycerine (dark cyan curves in Fig. 4a,b ). Previous works on patterned metal nanoparticle arrays have demonstrated comparable or even smaller linewidths from ~10 down to ~5 nm (refs 19 , 20 , 21 ), but the involved dips are in the spectral region shorten than ~950 nm. The spectral position of D1 versus the refractive index is plotted in Fig. 4c . A high refractive index sensitivity of 1,015 nm RIU −1 or 0.75 eV RIU −1 is obtained from linear fitting. FOM is a widely accepted metric for characterizing the performance of a refractive index sensor. The FOM value of our GMRA is determined to be 80–108, which is extremely high in comparison with those of LSPR-related sensors. This FOM is even comparable to the theoretically estimated upper limit (~108) for standard PSPR sensors made of gold under the Kretschmann configuration [37] , [38] . 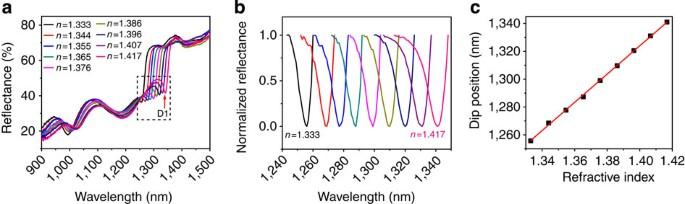Figure 4: Refractive index sensing using the GMRA. (a) Reflectance spectra of the GMRA immersed in glycerine−water mixture solutions with varying compositions at the incidence angle of 33.3°. (b) Normalized reflectance spectra for D1 in the spectral region indicated with the dashed box ina. (c) Relationship between the wavelength of D1 (solid squares) and the refractive index. The line is a linear fit, with the refractive index sensitivity and FOM value determined to be 1,015 nm RIU−1and 80−108, respectively. The standard deviation (s.d.) for all the data points (~0.2 nm) is too small to be seen. The sizes of the GMRA area=610 nm,h=510 nm,l=285 nm andt=110 nm. Figure 4: Refractive index sensing using the GMRA. ( a ) Reflectance spectra of the GMRA immersed in glycerine−water mixture solutions with varying compositions at the incidence angle of 33.3°. ( b ) Normalized reflectance spectra for D1 in the spectral region indicated with the dashed box in a . ( c ) Relationship between the wavelength of D1 (solid squares) and the refractive index. The line is a linear fit, with the refractive index sensitivity and FOM value determined to be 1,015 nm RIU −1 and 80−108, respectively. The standard deviation (s.d.) for all the data points (~0.2 nm) is too small to be seen. The sizes of the GMRA are a =610 nm, h =510 nm, l =285 nm and t =110 nm. Full size image GMRA as a label-free biosensor To demonstrate the application of the GMRA as plasmonic biosensors, GMRAs with a pillar height of h =480 nm were employed to detect Cyt c and AFP through nonspecific and specific interactions, respectively. The reflectance measurements for the detection were performed in a dry state. Compared with measurements in liquids, measurements in air are more convenient and sensitive because index changes caused by molecular adsorption are larger in air than in liquids. As the surrounding medium is changed from air to water, D1 shifts from the blue to red side of D4, as indicated by a similar array with h =510 nm. The entire spectral range covered by D1 can be well fitted linearly ( Supplementary Fig. S5 ), which is also in agreement with the linear dependence of WA position on the index at a fixed incidence angle. Cyt c is an electron-carrying protein and has a central role in cellular oxidation reactions in animals and plants. It has been extensively studied as a model system for biosensors [39] . The representative reflectance spectra measured when the array was exposed to Cyt c solutions at varying concentrations are shown in Fig. 5a . After each exposure, the array surface can be regenerated ( Supplementary Fig. S6 ). The adsorption and regeneration process is limited to 3–10 times depending on different arrays. 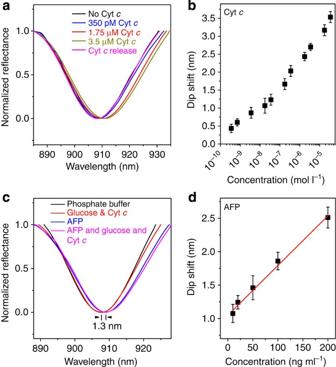Figure 5: Cytcand AFP detection. (a) Representative reflectance spectra of the same GMRA after the treatment of Cytcsolutions at different concentrations. The array surface was regenerated after the adsorption at each concentration. The spectrum (black) recorded without any Cytctreatment and that (pink) acquired after the regeneration from the adsorption at 3.5 μM are provided for reference. (b) Relationship between the shift of the dip and Cytcconcentration. (c) Reflectance spectra measured when an anti-AFP-functionalized GMRA was immersed in phosphate buffer (pH=7.1) without AFP, a mixture solution of glucose (5 mM) and Cytc(1.75 μM), an AFP solution (20 ng ml−1), and a mixture solution of AFP (20 ng ml−1), glucose (5 mM) and Cytc(1.75 μM), respectively. (d) Relationship between the shift of the dip and AFP concentration. The red line is a linear fit. The error bars inbanddrepresent s.d. calculated from three data points measured at each concentration. The sizes of the arrays are alla=610 nm,h=480 nm,l=265 nm andt=110 nm. Figure 5b shows the variation of the spectral position of the dip against Cyt c concentration. The red shift of the dip ranges from 0.4 to 3.5 nm as Cyt c concentration is increased from 350 pM to 35 μM. The detection limit of the GMRA sensor for Cyt c is estimated to be 200 pM. Figure 5: Cyt c and AFP detection. ( a ) Representative reflectance spectra of the same GMRA after the treatment of Cyt c solutions at different concentrations. The array surface was regenerated after the adsorption at each concentration. The spectrum (black) recorded without any Cyt c treatment and that (pink) acquired after the regeneration from the adsorption at 3.5 μM are provided for reference. ( b ) Relationship between the shift of the dip and Cyt c concentration. ( c ) Reflectance spectra measured when an anti-AFP-functionalized GMRA was immersed in phosphate buffer (pH=7.1) without AFP, a mixture solution of glucose (5 mM) and Cyt c (1.75 μM), an AFP solution (20 ng ml −1 ), and a mixture solution of AFP (20 ng ml −1 ), glucose (5 mM) and Cyt c (1.75 μM), respectively. ( d ) Relationship between the shift of the dip and AFP concentration. The red line is a linear fit. The error bars in b and d represent s.d. calculated from three data points measured at each concentration. The sizes of the arrays are all a =610 nm, h =480 nm, l =265 nm and t =110 nm. Full size image AFP was chosen to demonstrate that our GMRA is also applicable for relatively more complex biosensing applications where specific interactions are involved. AFP is a biomarker for hepatocellular carcinoma and germ cell tumours. The concentration of AFP in plasma is normally below 20 ng ml −1 but it increases markedly during the disease state [40] . Figure 5c shows the reflectance spectra measured when an anti-AFP-functionalized GMRA was incubated in the phosphate buffer, a mixture solution of glucose and Cyt c , an AFP solution (20 ng ml −1 ) and a mixture solution of AFP (20 ng ml −1 ), glucose and Cyt c , respectively. A red shift of 1.3 nm was detected for the dip only after the GMRA was exposed to AFP, and no shift was detected when the GMRA was immersed in the mixture solution of glucose and Cyt c before exposure to AFP ( Supplementary Fig. S7 ). In addition, the immersion of the GMRA in the mixture solution of AFP, glucose and Cyt c did not cause any further detectable shift, suggesting that AFP adsorption is close to saturation, and that nonspecific binding of glucose and Cyt c at high concentrations is suppressed. The shift of the dip increases from 1.1 to 2.5 nm as AFP concentration is raised from 10 ng ml −1 to 200 ng ml −1 ( Fig. 5d ). The detection limit for AFP is estimated to be 15 ng ml −1 . These results suggest that our GMRA offers a state-of-the-art system for label-free optical biosensing. We fabricated a GMRA structure, studied its plasmon modes and characterized its refractive index-sensing capabilities. The coupling of WA and the LSPRs in the array structure endows the GMRA with a very high FOM up to ~108, which is very close to the theoretically predicted upper limit for standard PSPR sensors made of gold films. Such a high FOM is mainly caused by the narrow FWHM, which is in turn induced by the Fano-type resonance arising from the interference between WA and the LSPRs supported by the gold caps and holes at the oblique incidence. To more clearly ascertain the plasmon modes of the GMRA, we further measured the reflectance spectrum of the GMRA in water at normal incidence and compared it with those simulated for the GMRA, the sole gold film with the periodic holes filled with the photoresist pillars, and the sole periodic array of the photoresist pillars with the gold caps in water at normal incidence ( Fig. 6 ). The LSPR arising from the gold caps is centred at 1,053 nm ( Fig. 6c , P1′). Its FWHM is very broad, with a value of ~500 nm. In comparison, the LSPR arising from the gold holes is centred at 1,174 nm ( Fig. 6a , D4′). The dip (D4) caused by the LSPR of the gold holes is located within the broad LSPR peak (P1) of the gold caps. Therefore, similar to the case in air, the dip around 1,290 nm on the reflectance spectrum of the GMRA in water results from the interference of the LSPRs of the gold holes and caps ( Fig. 6b ). The assignment of the LSPRs is confirmed by the simulated electric field intensity distributions at the peaks and dips ( Fig. 6d–g ). In addition, the dip around 840 nm on the spectrum of the GMRA in water is confirmed to be (1, 0) WA. As the incidence angle is increased, (1, 0) WA in water shifts to the longer-wavelength region. It eventually overlaps with the dip around 1,290 nm when the incidence angle is increased above ~30° ( Fig. 7a ). As a result, a dip with a Fano-like lineshape is produced through the interference between (1, 0) WA and the LSPRs of the gold holes and caps in water ( Fig. 7b ). The electric field at this Fano-like dip is mainly localized at the gold caps and holes ( Fig. 7c ), whereas that at the rapidly raised shoulder on the right side of the dip is dominated by the LSPR of the gold caps ( Fig. 7d ). The extremely narrow Fano-like dip is believed to be the main reason for the GMRA to have such a high FOM. The lifted gold mushroom caps give rise to an increased apparent refractive index sensitivity, which also has a role in the increase of the FOM. We also note that because the sensor is based on the coupled WA–LSPR mode, the spectral range for detection and the targeted index range can both be readily tailored by adjusting the geometrical parameters, that is, the lattice constants and pillar sizes, to shift the anticrossing point between WA and the LSPRs. 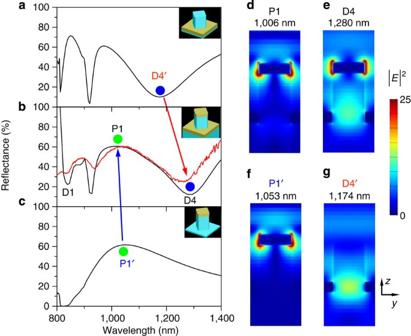Figure 6: Reflectance and electric field intensity distributions of various structures at normal incidence in water. (a) Simulated reflectance spectrum for the structure composed of only the photoresist pillars and perforated gold film. (b) Measured (red curve) and simulated (black curve) reflectance spectra for the GMRA (a=610 nm,h=510 nm,l=285 nm andt=110 nm). (c) Simulated reflectance spectrum for the structure composed of only the periodic array of the gold mushrooms but without the perforated gold film. The insets ina–care the schematics of the simulated structures. The red arrow indicates that the dip D4 inband the dip D4′ inahave a similar origin, and the blue arrow indicates that the peak P1 inband the peak P1′ inchave the same origin. (d–g) Simulated electric field intensity distributions at the indicated peak and dip positions at the linear scale. Figure 6: Reflectance and electric field intensity distributions of various structures at normal incidence in water. ( a ) Simulated reflectance spectrum for the structure composed of only the photoresist pillars and perforated gold film. ( b ) Measured (red curve) and simulated (black curve) reflectance spectra for the GMRA ( a =610 nm, h =510 nm, l =285 nm and t =110 nm). ( c ) Simulated reflectance spectrum for the structure composed of only the periodic array of the gold mushrooms but without the perforated gold film. The insets in a – c are the schematics of the simulated structures. The red arrow indicates that the dip D4 in b and the dip D4′ in a have a similar origin, and the blue arrow indicates that the peak P1 in b and the peak P1′ in c have the same origin. ( d – g ) Simulated electric field intensity distributions at the indicated peak and dip positions at the linear scale. 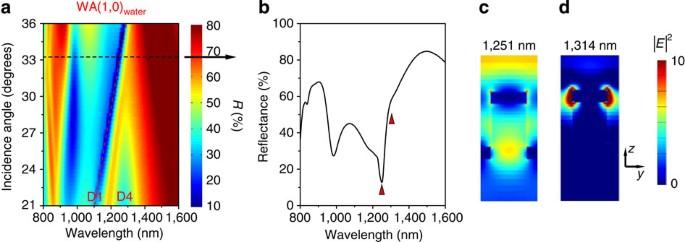Figure 7: Angle-resolved reflectance spectra of the GMRA immersed in water. (a) Simulated reflectance spectra with the incidence angle varied from 21° to 36°. The red dashed line denotes (1, 0) WA. (b) Simulated reflectance spectrum for the incidence angle of 33.3°, as indicated by the black dashed line ina. (c) Electric field intensity distributions at 1,251 and 1,314 nm, respectively, as indicated by the solid triangles inb, at the linear scale. The sizes of the GMRA area=610 nm,h=510 nm,l=285 nm andt=110 nm. Full size image Figure 7: Angle-resolved reflectance spectra of the GMRA immersed in water. ( a ) Simulated reflectance spectra with the incidence angle varied from 21° to 36°. The red dashed line denotes (1, 0) WA. ( b ) Simulated reflectance spectrum for the incidence angle of 33.3°, as indicated by the black dashed line in a . ( c ) Electric field intensity distributions at 1,251 and 1,314 nm, respectively, as indicated by the solid triangles in b , at the linear scale. The sizes of the GMRA are a =610 nm, h =510 nm, l =285 nm and t =110 nm. Full size image In our determination of the refractive index sensitivity of the GMRA, the index changes are large ( Fig. 4 ). Such large index changes do not suggest that our GMRA has a limited sensing resolution. The index change in each step is determined by the angle adjustment resolution (0.5°) of our spectrophotometer because the incidence angle from the solution to the GMRA needs to be kept unchanged during the measurements by adjusting the incidence angle from air to the solution. We estimated the resolution of our GMRA by keeping the incidence angle from air to the solution unchanged and varying the solution index slightly ( Supplementary Fig. S8 ). At the spectral resolution (0.1 nm) of our spectrophotometer, the estimated sensing resolution is ~2 × 10 −4 RIU. If the spectral resolution of the optical detection system can be improved to 0.01 nm, the sensing resolution of our GMRA can be increased to 10 −5 RIU. The sensing resolutions of our GMRA are comparable to those of PSPR sensors reported previously [38] , [41] . Compared with commercial PSPR systems with sensing limitations of 10 −7 RIU, although the FOM of our GMRA sensor is close to the theoretically predicted FOM limit for standard PSPR sensors under the Kretschmann configuration, the optical detection system and manner (wavelength or intensity) have to be optimized to achieve the best sensing resolution. We also note that a closely related array structure has been reported recently, which consists of periodically perforated nanoscale holes in a gold film with a gold nanodisk at the bottom of each hole [42] , [43] , [44] . This structure can be thought of as an inverse one to our GMRA. The sensing mechanisms of these two types of array structures are very different. The sensing of the reported structure is based on the interference between WA and the PSPR of the upper perforated gold film. In our GMRA, the gold caps are on the top of the photoresist pillars, which induces a strong LSPR. The sensing of our GMRA relies on the interference between the LSPRs and WA. The coupled resonance mode has a very narrow FWHM, giving rise to a very high FOM. In summary, we have designed and fabricated a periodic array of gold mushrooms, each of which is made up of a gold cap on the top, a photoresist pillar and a hole in a gold film at the bottom. The gold caps supported on the pillars have more surface regions accessible by the surrounding environment, and the periodic array gives rise to a Fano resonance between the LSPR and WA. The narrow spectral linewidth caused by the Fano resonance together with the increased apparent index sensitivity enables the GMRA to possess a FOM reaching the theoretical upper limit of PSPR sensors. We have further demonstrated the GMRA as a plasmonic biosensor for detecting Cyt c and AFP, with their detection limits down to 200 pM and 15 ng ml −1 , respectively. The GMRA is fabricated by double two-beam lithography and thermal evaporation of gold. The two-step fabrication is simple and cost-effective, which will facilitate the widespread applications of the GMRA in label-free chemical and biomedical sensing. GMRA fabrication The fabrication procedure is schematically shown in Fig. 1a . A thin film of PMMA (molecular weight (MW): 350,000, 1.5 wt% in chlorobenzene) was first spin-coated on a cleaned quartz slide at 4,000 r.p.m. for 35 s. The PMMA film functioned as an adherent to ensure the firm attachment of the photoresist pillars. The PMMA film was treated on a hot plate at 180 °C for 5 min to evaporate chlorobenzene. Its thickness was ~50 nm. A positive photoresist (AR 3740, Allresist) film was then spun onto the PMMA film at 2,000 r.p.m. for 35 s from a 14.5-wt% solution in a thinner (AR 300-12, Allresist). The photoresist film was baked at 95 °C for 2 min. Its thickness was 480–530 nm owing to the fluctuation in the humidity in the lab. The photoresist film was thereafter subjected to double exposure under an interference pattern of two continuous laser beams (457.9 nm). The incidence angles of the two laser beams on the photoresist film were ±22° and the laser power on the film was 30 mW for each. The two exposures were orthogonal to each other. Each exposure lasted for 18 s. After the exposures, the photoresist film was immersed in a developer (AR 300-26, Allresist) at 21 °C for 35 s to give a photoresist pillar array in a square lattice. The GMRA was finally obtained after sequential thermal evaporation of 5-nm nickel and 110-nm gold on the photoresist array. Measurements of the reflectance spectra All zero-order reflectance spectra were taken on a ultraviolet/visible/near-infrared spectrometer (Lambda 950, PerkinElmer) under s -polarized incident waves, with the electric field perpendicular to the incidence plane. The incidence angle of the spectrometer can be changed from 8° to 68° at an accuracy of 0.5°. For recording the reflectance spectra at normal incidence, one beam splitter and three silver mirrors were placed in the optical path, as shown schematically in Supplementary Fig. S9 . All reflectance spectra were corrected by dividing them with the reflectance spectrum of a silver mirror, which served as a reference only. A Glan–Taylor prism was employed in the optical path to generate polarized incident waves. Refractive index sensitivity measurements The index sensitivity was determined by immersing the same GMRA in different glycerine–water mixture solutions and measuring the reflectance spectra. To keep the incidence angle at a constant value in different mixture solutions, we adjusted the incidence angle in air according to Snell’s law n air sin θ air = n sol sin θ sol . To obtain the incidence angle from the solution to the array surface at 33.3°, the concentrations of glycerine were chosen to be 0, 9.33, 17.85, 25.96, 33.74, 41.46, 48.86, 55.75 and 62.50 wt%, and the corresponding refractive indices were 1.333, 1.344, 1.355, 1.365, 1.376, 1.386, 1.396, 1.407 and 1.417, respectively. After each measurement, the array was rinsed carefully with deionized water. After the rinsing process, the dip was found to return to approximately the same spectral position as that measured in water in the beginning ( Supplementary Fig. S10 ). To determine the s.d. of the dip position at each refractive index, the array was immersed in the mixture solvent. After the reflectance spectrum was recorded, the array was taken out, rinsed with water and dried with flowing nitrogen. This procedure was repeated and three measurements were made at each refractive index. Cyt c and AFP detection An ethanolic solution of 11-mercaptoundecanoic acid (20 mM) was first spin-coated on a flat poly(dimethylsiloxane) stamp. After drying, the poly(dimethylsiloxane) stamp was sealed on the GMRA for 30 s and peeled off. The GMRA was then soaked in a mixture solution of 3-mercaptopropionic acid and 6-mercapto-1-hexanol at a molar ratio of 5:1 in phosphate buffer (2 mM in total) for 12 h. These treatments ensured that the entire gold surface of the array was covered by a self-assembled monolayer containing pendent hydrophilic groups via covalent thiol chemistry. The unreacted thiol molecules were washed away by phosphate buffer (pH=7.1) and deionized water. For Cyt c detection, the surface-functionalized GMRA was covered in an area of 10 × 10 mm 2 with 100 μl of Cyt c (from horse heart, MW=~13 kDa, p K a=~9.6) dissolved in phosphate buffer (pH=7.1). After the solution was kept on the array for 1 h, the array was washed with phosphate buffer (pH=7.1) and deionized water, and was then dried. The reflectance spectrum was measured at an incidence angle of 30°. To regenerate the surface of the GMRA, the adsorbed Cyt c molecules were released from the gold surface by rinsing the array first with phosphate buffer (pH=2.1) and then with deionized water. Under the acidic environment, the mercaptoalkyl acids were neutral, which caused the release of the Cyt c molecules during rinsing. The surface regeneration was checked by the spectral measurements. The adsorption and regeneration process could be repeated 3–10 times for different arrays. For the concentration-dependent measurements, multiple arrays were fabricated under the same conditions, with each array for one concentration. The spectral positions of D1 measured in air at the incidence angle around 30° varied within 10 nm among the different arrays. At each concentration, after Cyt c adsorption, the spectral measurements were repeated three times, where the array was taken off the spectrophotometer, rinsed with phosphate buffer (pH=7.1) and water, dried with flowing nitrogen and mounted on the spectrophotometer again at each time. For AFP (Fapon Biotech Inc., Shenzhen, China) detection, the surface-functionalized GMRA was further treated with an AFP antibody (anti-AFP, Fapon Biotech Inc.) through covalent binding. Twenty microlitres of freshly prepared solution containing carbodiimide hydrochloride (400 mM) and N -hydroxysuccinimide (100 mM) were placed on the GMRA surface and washed off after 30 min, which was followed immediately by a 2-h incubation at room temperature with 20 μl of anti-AFP (1.0 mg ml −1 ) in phosphate buffer (pH=7.1). After being washed with the buffer, the GMRA was further incubated in an aqueous 6-mercapto-1-hexanol solution (0.2 vol%) for 40 min to block the excess active groups and nonspecific-binding sites on the surface. After the GMRA was washed with the buffer and dried, its reflectance spectrum was measured and the dip position was recorded as the reference. To detect AFP, the GMRA functionalized with anti-AFP was covered with 100 μl of AFP (MW=~69 kDa) dissolved in phosphate buffer (pH=7.1). After 30 min, when AFP adsorption reached equilibrium, the array was washed thoroughly with the buffer and deionized water, and was then dried. The concentration-dependent measurements were carried out using different arrays fabricated under the same conditions. The detection selectivity for AFP was examined by comparing the reflectance spectra measured when an anti-AFP-functionalized GMRA was incubated, respectively, in phosphate buffer (pH=7.1), a mixture solution of glucose (5 mM) and Cyt c (1.75 μM), an AFP solution (20 ng ml −1 ), and a mixture solution of AFP (20 ng ml −1 ), glucose (5 mM) and Cyt c (1.75 μM). At each step, the GMRA was washed thoroughly with the buffer and deionized water and then dried before the reflectance measurement. For the estimation of the detection limits, the data points of the concentration-dependent shifts of D1 were linearly fitted with Δ λ =Δ λ 0 + Sc , where Δ λ is the dip shift, Δ λ 0 is the intercept on the shift axis, S is the slope and c is the concentration. If the s.d. obtained from the fitting for Δ λ 0 is σ , then the detection limit c limit can be estimated according to c limit =3 σ / S . As the concentration is plotted at the logarithmic scale for Cyt c , 10 −10 M was taken as the zero point of the concentration axis. Only the first five points were used for linear fitting against the logarithmic values of Cyt c concentrations. FDTD simulations The simulations were performed using a commercial software (FDTD solutions, Lumerical Solutions) to generate the reflectance spectra and electric field distributions of the GMRA at normal and oblique incidences. The structure was excited with s -polarized plane-wave light. Bloch boundary conditions were applied in both x and y axes. A mesh size of 4 nm for the metal region was utilized. The dielectric functions of bulk gold in the near-infrared region were described according to the Drude model with the plasma frequency ω pl =1.37 × 10 16 rad s −1 and the damping frequency ω damp =7.536 × 10 14 rad s −1 . The used refractive indices for the photoresist, PMMA and quartz were 1.6, 1.49 and 1.48, respectively. Each unit in the array was modelled as a rounded square gold cap supported on a photoresist pillar with straight side walls. All the sizes were set according to the measured ones from the SEM images. We also performed FDTD simulations by modelling the gold caps as circular and unrounded square ones and by using the dielectric function of gold from Johnson and Christy ( Supplementary Figs S11 and S12 ). The calculated reflectance spectra for rounded square caps and with the dielectric function of gold based on the Drude model are found to be closer to the experimental ones. How to cite this article: Shen, Y. et al . Plasmonic gold mushroom arrays with refractive index sensing figures of merit approaching the theoretical limit. Nat. Commun. 4:2381 doi: 10.1038/ncomms3381 (2013).